Glycopeptide analogues of PSGL-1 inhibit P-selectinin vitroandin vivo Blockade of P-selectin (P-sel)/PSGL-1 interactions holds significant potential for treatment of disorders of innate immunity, thrombosis and cancer. Current inhibitors remain limited due to low binding affinity or by the recognized disadvantages inherent to chronic administration of antibody therapeutics. Here we report an efficient approach for generating glycosulfopeptide mimics of N-terminal PSGL-1 through development of a stereoselective route for multi-gram scale synthesis of the C2 O-glycan building block and replacement of hydrolytically labile tyrosine sulfates with isosteric sulfonate analogues. Library screening afforded a compound of exceptional stability, GSnP-6, that binds to human P-sel with nanomolar affinity ( K d ~22 nM). Molecular dynamics simulation defines the origin of this affinity in terms of a number of critical structural contributions. GSnP-6 potently blocks P-sel/PSGL-1 interactions in vitro and in vivo and represents a promising candidate for the treatment of diseases driven by acute and chronic inflammation. The vascular endothelium forms a dynamic interface between blood elements and peripheral tissues. Characteristically, leukocyte–endothelial interactions are mediated by transient tethering, followed by rapid integrin activation and subsequent transendothelial migration [1] , [2] . The recruitment of leukocytes to sites of inflammation is mediated by selectin adhesion molecules and their ligands [3] . P-selectin (P-sel) [4] , [5] , found on activated platelets and vascular endothelium, is rapidly translocated to the cell surface within minutes of an inflammatory stimulus, E-sel [6] is expressed on endothelial cells after de novo synthesis within a few hours of activation, while L-sel is expressed on most leukocytes and functions as a homing receptor to mediate binding of lymphocytes to high endothelial venules of peripheral lymph nodes [7] . Excessive trafficking of leukocytes to extravascular locations can lead to tissue injury contributing to the development of inflammatory bowel disease, chronic obstructive pulmonary disease, atherosclerosis and post-thrombotic syndrome, among a variety of other disorders. Thus, selectins, as a mediator of early adhesion and intracellular signalling events in the inflammatory cascade, represent a promising target for the design of agents that limit adverse inflammatory responses. While structurally diverse glycoprotein counter-receptors bind selectins with high affinity, the most well characterized ligand is P-sel-glycoprotein-ligand-1 (PSGL-1) [8] . PSGL-1 binds all three selectins, but with highest affinity to P-sel [9] . Ligation of P-sel expressed on endothelial cells by PSGL-1 constitutes the initial ‘capture and rolling’ step in the leukocyte–endothelial cell adhesion cascade [10] . Likewise, the interaction of PSGL-1 with P-sel on activated platelets promotes formation of leukocyte–platelet aggregates that contributes to adhesion and infiltration of inflammatory cells and both activated platelets and soluble P-sel promote leukocyte infiltration [11] , [12] , [13] . Significantly, the engagement of PSGL-1 to P-sel activates intracellular signalling pathways that induces the β2-integrin LFA-1 to adopt an extended conformation associated with the intermediate affinity state, which supports leukocyte deceleration and cell arrest onto the endothelium [14] . PSGL-1 also activates the expression of intracellular protein kinases, such as Rho/Rock kinase, which mediates cell migration, and MAPK kinase that controls expression of pro-inflammatory cytokines [15] , [16] . Blockade of P-sel/PSGL-1 interactions holds significant potential for the treatment of disorders due to maladaptive acute or chronic inflammatory responses [17] , [18] , [19] . The role of P-sel/PSGL-1 in a number of disease states has led to the design of a variety of biologics, small molecules and glycopeptide mimics to target these interactions. Although P-sel and PSGL-1 blocking antibodies are undergoing clinical evaluation for the treatment of sickle cell disease and Crohn’s disease, they are expensive to manufacture, limited in shelf-life and the development of antibodies against monoclonal therapeutics, including chimeric and humanized monoclonal antibodies, continues to limit the effectiveness of antibody therapy especially when there is need for daily or long-term administration [20] . Small molecule inhibitors designed through modifications of sialyl Lewis x (sLe x ) continue to be limited by their low potency and off-target toxicity. For example, GMI-1070 has demonstrated efficacy in treating sickle cell disease, but its low activity to P-sel (IC 50 ~423 μM) requires infusion of ~2 g of drug per day [21] . Likewise, PSI-697 only weakly inhibits human platelet–monocyte aggregation, which is almost certainly attributable to its low K d ~200 μM (ref. 22 ). Similarly, the glycomimetic, bimosiamose (TBC1269), is a pan-sel inhibitor with an IC 50 of 70 μM against P-sel and an IC 50 of >500 μM against E- and L-sel [23] . Most existing P-sel inhibitors have been designed to mimic the core-2 O -glycan (C2 O -glycan) bearing sLe x moiety, but often fail to account for the crucial contributions of multiple clustered tyrosine sulfates [21] , [24] , [25] . Indeed, Leppänen et al. [26] , [27] , [28] have shown that high affinity binding of P-sel to PSGL-1 requires stereospecific interactions with both clustered tyrosine sulfates (Tyr-SO 3 H) and a nearby C2 O -glycan bearing a sLe x -containing hexasaccharide epitope (C 2 - O -sLe x ). To date, attempts to synthesize mimics of the N terminus of PSGL-1 have been limited by the acid sensitivity of tyrosine sulfates [29] , [30] , poor selectivity in key glycosylation steps [31] and incompatible protecting groups for oligosaccharide synthesis [32] . We report an efficient approach for the generation of a diverse set of glycopeptide mimics of PSGL-1. Key features of this synthesis include an efficient stereoselective route that has lead to multi-gram scale synthesis of the C2 O -glycan and replacement of hydrolytically labile tyrosine sulfates with stable, isosteric sulfonate analogues affording compounds with high affinity to P-sel ( K d 14–22 nM). In the process, we identified a high affinity, chemically stable compound, termed GSnP-6 that blocks PSGL-1/P-sel interactions in vitro and in vivo . Compound design and strategy In our approach, we envisaged a building block containing protecting groups fully compatible with peptide synthesis, after which sLe x would be incorporated. Appendages were selected so that the resulting compounds could be selectively extended by glycosyltransferases to provide a diverse array of glycopeptide mimetics of PSGL-1. In this regard, we previously identified a threonine-derived C2 O -glycan as an appropriate building block for such studies [33] . However, attempts to synthesize the glycoamino acid building block suffered from suboptimal regioselectivity ( α / β : 1:2:6) in the key glycosylation step. Furthermore, use of a glycosyl imidate donor required a triflic azide-mediated diazotransfer step, which is potentially explosive, thus prohibiting deployment of this scheme for preparative scale synthesis (>50 g). As a result, the C2 O -glycan was only obtained on milligram scale. To circumvent these problems, a more efficient scheme was developed that lead to multi-gram scale synthesis of this key compound. Synthesis began from 3,4,6 tri- O -acetyl-D-galactal, which can be readily converted to a halide via a one-pot azidochlorination step ( Fig. 1 ). Although previously reported [34] , direct coupling of the chloride intermediate with a Fmoc-threonine acceptor was unsuccessful due to its rapid decomposition. Therefore, this intermediate was converted in situ to the thioglycoside donor 1 . Significantly, this two-step, one-pot procedure could be safely carried out on a preparative scale (>50 g) to provide donor 1 in 67% yield. Azidochlorination does not completely eliminate explosive risk, but it is substantially reduced and greatly facilitates safe, large-scale production. Coupling with the Fmoc-threonine acceptor afforded 2 in 78% yield with high α selectivity ( α / β : 95:5). Glycoamino acid 2 was then converted to diol 5 by following previously reported steps [33] . Significantly, this new scheme provided acceptor 5 in less than seven steps with 21% overall yield, which established this route for this key building block as the most efficient and convenient to date [31] , [32] , [33] . 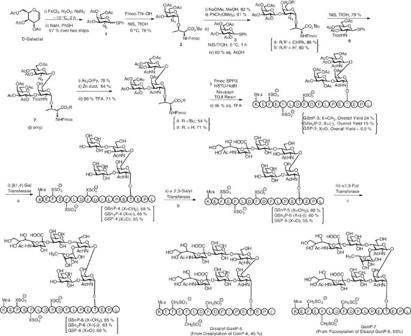Figure 1: Synthesis of the Core-2 glycan and subsequent enzymatic steps to afford a family of 17 glycopeptide mimetics of PSGL-1. Enzymatic steps (a) UDP-Gal, β-1,4-GalT (bovine), alkaline phosphatase, 130 mM HEPES, pH 7.4, 40 mM sodium cacodylate, pH 7.0, 20 mM MnCl2and 0.02% NaN3; (b) α 2,3-(N)-sialylT CMP-NeuAc 50 mM MOPS, pH 7.4, 0.1% bovine serum albumin and 0.02% NaN3, 14 h; (c) GDP-Fuc, α1,3-FucT-VI, 50 mM MOPS, pH 7.4, 20 mM MnCl2and 0.02% NaN3, 16 h. The desialylated GSnP-6 was obtained from GSnP-4 in 45% yield. GSnP-7 was obtained in 55% yield by fucosylation of disialylated GSnP-6. 4-(Sulfomethyl)phenylalanine series (n): GSnP-6 (X: CH2; R=H); GSnP-7 (X: CH2; R=Sialyl);4-(Sulfo)phenylalanine series (n2): GSn2P-6 (X: bond; R=H); Tyrosine O-sulfate series: GSP-6 (X: O; R=H). The last numeral refers to the size of the glycan (for example, 6 for hexasaccharide). Figure 1: Synthesis of the Core-2 glycan and subsequent enzymatic steps to afford a family of 17 glycopeptide mimetics of PSGL-1. Enzymatic steps ( a ) UDP-Gal, β-1,4-GalT (bovine), alkaline phosphatase, 130 mM HEPES, pH 7.4, 40 mM sodium cacodylate, pH 7.0, 20 mM MnCl 2 and 0.02% NaN 3 ; ( b ) α 2,3-( N )-sialylT CMP-NeuAc 50 mM MOPS, pH 7.4, 0.1% bovine serum albumin and 0.02% NaN 3 , 14 h; ( c ) GDP-Fuc, α1,3-FucT-VI, 50 mM MOPS, pH 7.4, 20 mM MnCl 2 and 0.02% NaN 3 , 16 h. The desialylated GSnP-6 was obtained from GSnP-4 in 45% yield. GSnP-7 was obtained in 55% yield by fucosylation of disialylated GSnP-6. 4-(Sulfomethyl)phenylalanine series ( n ): GSnP-6 (X: CH 2 ; R=H); GSnP-7 (X: CH 2 ; R=Sialyl); 4- (Sulfo)phenylalanine series ( n 2 ): GSn 2 P-6 (X: bond; R=H); Tyrosine O-sulfate series: GSP-6 (X: O; R=H). The last numeral refers to the size of the glycan (for example, 6 for hexasaccharide). Full size image In the key glycosylation step with acceptor 5 , we anticipated that the axial 4-OH group would be of low reactivity, especially when carrying a substituent at O-3. However, an undesired tetrasaccharide was identified in ~20% yield [33] . Both desired and undesired compounds had similar retention factor values. Thus, chromatographic separation was challenging and laborious, particularly at a preparative scale. To address this problem, we performed low temperature activation (−10 °C) with glucosamine donor 6 at 0.8 equiv. (as opposed to 1.2 equiv. ), which produced only the β-glycoside 7 in 79% yield ( Supplementary Figs 1 and 2 ). The (1→6)-linkage in 7 was confirmed by nuclear Överhauser enhancement spectroscopy (NOESY) spectrum, which displayed a cross-peak between H-1 of the glucosamine residue and H-6 of the galactosamine residue. gHMBC nuclear magnetic resonance (NMR) of 7 confirmed that O-6 was glycosylated in revealing cross-peaks from 101.3 p.p.m. (C-1 of the glucosamine residue, A-C1) and 4.02 p.p.m. (H-6 of the galactosamine residue, BH6), as well as from 4.70 p.p.m. (H-1 of the glucosamine residue, A-H1) and 69.5 p.p.m. (C-6 of the galactosamine residue, B-C6) ( Supplementary Figs 3–7 ). Acetylation of 7 with Py/Ac 2 O, zinc reduction and TFA-mediated t -butyl ester deprotection provided the C2 O -glycan 9 ( Supplementary Figs 8 and 9 ). This new route improved not only selectivity and yield, but also enabled the production of gram quantities of intermediate 9 and facilitated the synthesis of a broad range of structural mimics of PSGL-1. With the availability of this glycoamino acid building block, glycopeptide mimics of the N-terminal domain of PSGL-1 were synthesized using a Fmoc-assisted SPPS strategy ( Fig. 1 ). Coupling reactions were performed using 2-(1H-benzotriazole-1-yl)-1,1,3,3-tetramethyluronium hexafluorophosphate (HBTU) and 1-hydroxy-benzotriazol (HOBt) and the deprotection step was carried out with 20% piperidine. Addition of the sterically hindered C2 glycoamino acid 9 proceeded smoothly without formation of any side products. However, the incorporation of Fmoc-Tyr (O-SO 3 − ) amino acid in peptide synthesis is extremely challenging owing to its acid lability [35] . As an alternative approach, enzymatic sulfation has been proven less than ideal since tyrosine sulfotransferase is not commercially available, and while the enzymatic reaction is optimal at 30 °C tyrosine sulfotransferase is unstable >20 °C (ref. 36 ). Chemical sulfation of tyrosine residues after peptide synthesis also suffers from low specificity [30] , incomplete reaction with sulfating reagents [37] , and low yield [38] . Together, these factors place significant limitations on the use of Tyr (O-SO 3 − ), which has limited their broad application in drug design. Therefore, we elected to replace the acid labile Tyr (O-SO 3 − ) moiety with bioiosteric, hydrolytically stabile analogues, namely, Fmoc-Phe ( p -CH 2 SO 3 H) [39] , [40] and Fmoc-Phe ( p -SO 3 H) [41] . Such sulfonate mimics can be readily incorporated in solid phase peptide synthesis without the need for any side-chain protecting groups using standard HBTU coupling conditions. The chromogenic amino acid Fmoc-Lys(Mca)-OH was also incorporated at the N terminus of the PSGL-1 sequence for facile detection and quantification. After peptide synthesis, the deprotection of sulfonate mimics could be readily carried out with 95% aqueous TFA at room temperature. Saponification of O-acetate groups in GS (n) P-3 was achieved with catalytic NaOMe to afford the glycopeptide mimics, which were further purified by reversed-phase high-performance liquid chromatography (RP-HPLC). In synthesizing the native tyrosine O-sulfate sequence, glycosulfopeptide-3 (GSP-3), deprotection was performed at 0 °C to suppress the degradation of tyrosine O-sulfates [42] . When tyrosine O-sulfates were employed in peptide synthesis, overall yield of GSP-3 was <0.5%, indicating the labile nature of tyrosine sulfates [36] , [43] . In contrast, use of hydrolytically stable tyrosine sulfonate analogues resulted in a dramatic improvement in overall yield to afford GSnP-3 and GSn 2 P-3 in 24% and 19% yields, respectively. The sLe x moiety was incorporated into GS (n) P-3 by using glycosyltransferases in stepwise order to sequentially add galactose, sialic acid and fucose. The highly efficient β1,4-galactosyltransferase (β1,4-GalT) is commercially available and was used to initially install β1,4-galactose. Since sialyltransferases have low efficiency towards a fucosylated Le x structure, fucose was installed after sialylation. Thus, galactose was first appended in a β1,4 linkage to GlcNAc by treatment with β1,4-GalT in the presence of UDP-Galactose to produce GS(n)P-4. Similarly, addition of sialic acid was achieved by incubation of GSnP-4 with α2,3-sialyltransferase (α,2,3-(N)-sialylT) in the presence of CMP-NeuAc to obtain GSnP-5. The sLe x structure was completed by incubation of GS (n) P-5 with human α1,3-fucosyltransferase V and GDP-Fucose to produce GS (n) P-6. All enzymatic steps proceeded with 60 to 70% yield without observed interference of the sulfonate residues [44] . In addition, desialylated glycopeptide mimics were generated through additional sialylation of GSnP-4 to provide disialyl GSnP-6 (45% yield) followed by fucosylation to provide GSnP-7 in 55% yield. Using this approach, a diverse array of 17 glycopeptide mimics of PSGL-1 was synthesized including GSnP[3–6], disialyl GSnP-6, GSnP-7, GSn 2 P[3–6], GSP[3–6] and three GSnP C1 peptides ( Fig. 1 , Supplementary Figs 10–17 ). GSnP-6 demonstrates nanomolar affinity to P-sel The binding affinity of this set of glycopeptide mimics towards P-, L- and E-sel was initially screened using microarray technology. The 17 glycopeptide mimics along with five glycan standards (sLe x , NA2, NA2,3, NA2,6 and LNnT) were printed on a NHS-activated glass slide. The slide was then incubated with recombinant immunoglobulin (Ig) chimeras of P-, L- or E-sel (5–20 μg ml −1 ) followed by Alexa-488-labelled anti-human IgG antibody (5 μg ml −1 ). Similar to the native, N-terminal PSGL-1 sequence containing tyrosine sulfate (GSP-6), GSnP-6 bound to P-sel more strongly than to E- or L-sel ( Fig. 2a–c , Supplementary Fig. 18 ). Likewise, GSnP-7, a sialylated extension of GSnP-6, showed higher affinity to P-sel. However, disialyl GSnP-6, lacking the fucosyl residue displayed lower affinity to P-sel, consistent with the key contribution of α1,3-fucose. Binding of glycopeptide mimics was Ca 2+ dependent and inhibited by EDTA. 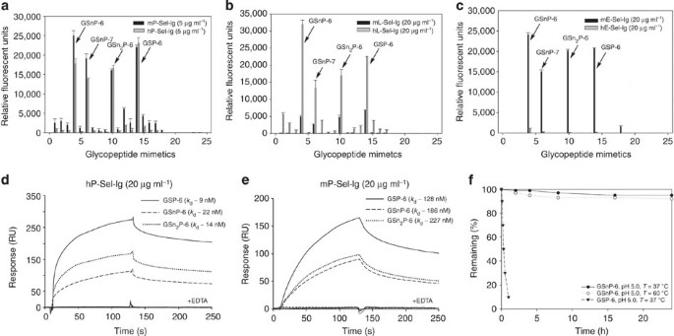Figure 2: Binding of P-, E- or L-selectin to PSGL-1 glycopeptide mimics and GSnP-6 stability analysis. Microarray binding studies of glycopeptide mimics towards (a) human and mouse P-selectin (5 μg ml−1), (b) human and mouse L-selectin (20 μg ml−1) and (c) human and mouse E-selectin (20 μg ml−1). The compounds printed on the microarray in the order depicted here ina–care detailed inSupplementary Fig. 18. Reference compounds included sialyl Lewis x (sLex), the biantennary glycans NA2, NA2,3, NA2,6, as well as lacto-N-neo-tetraose (LNnT) and biotin. Bound selectin-Igs were detected using Alexa-488-labelled anti-human IgG antibody (5 μg ml−1). Three lectins RCA-1, AAL and PNA were used to confirm the sequence of enzymatic steps. Monoclonal antibodies CHO131, PSG2 antibody and PL-1 were used to confirm the presence of sLex, tyrosine sulfates and the peptide sequence, respectively. Biacore binding analysis to human P-selectin with observed rate constants for (d) GSnP-6,kon3.1 × 105M−1s−1,koff6.9 × 103s−1; GSn2P-6,kon6.4 × 105M−1s−1,koff6.8 × 103s−1. Biacore binding analysis tomouseP-selectin with observed rate constants for (e) GsnP-6,kon4.9 × 104M−1s−1,koff8.0 × 103s−1; GSn2P-6kon5.3 × 104M−1s−1,koff9.0 × 103s−1. (f) Temperature- and pH-dependent stability studies of GSnP-6. Figure 2: Binding of P-, E- or L-selectin to PSGL-1 glycopeptide mimics and GSnP-6 stability analysis. Microarray binding studies of glycopeptide mimics towards ( a ) human and mouse P-selectin (5 μg ml −1 ), ( b ) human and mouse L-selectin (20 μg ml −1 ) and ( c ) human and mouse E-selectin (20 μg ml −1 ). The compounds printed on the microarray in the order depicted here in a – c are detailed in Supplementary Fig. 18 . Reference compounds included sialyl Lewis x (sLe x ), the biantennary glycans NA2, NA2,3, NA2,6, as well as lacto- N -neo-tetraose (LNnT) and biotin. Bound selectin-Igs were detected using Alexa-488-labelled anti-human IgG antibody (5 μg ml −1 ). Three lectins RCA-1, AAL and PNA were used to confirm the sequence of enzymatic steps. Monoclonal antibodies CHO131, PSG2 antibody and PL-1 were used to confirm the presence of sLe x , tyrosine sulfates and the peptide sequence, respectively. Biacore binding analysis to human P-selectin with observed rate constants for ( d ) GSnP-6, k on 3.1 × 10 5 M −1 s −1 , k off 6.9 × 10 3 s −1 ; GSn 2 P-6, k on 6.4 × 10 5 M −1 s −1 , k off 6.8 × 10 3 s −1 . Biacore binding analysis to mouse P-selectin with observed rate constants for ( e ) GsnP-6, k on 4.9 × 10 4 M −1 s −1 , k off 8.0 × 10 3 s −1 ; GSn 2 P-6 k on 5.3 × 10 4 M −1 s −1 , k off 9.0 × 10 3 s −1 . ( f ) Temperature- and pH-dependent stability studies of GSnP-6. Full size image Dissociation constants ( K d ) were determined using a Biacore binding assay after initial capture of biotinylated GS (n) P-6 onto streptavidin-coated sensor chips followed by flow through of P-, L- or E-sel-Ig (2.5–60 μg ml −1 ). Dissociation constants for GSnP-6 and GSn 2 P-6 to human P-sel were 22 and 14 nM ( Fig. 2d ), respectively, compared with the reported K d of 73 nM for native PSGL-1 (ref. 9 ). The K d of GSnP-6 to murine P-sel was approximately ninefold lower than to human P-sel ( Fig. 2e ). GSnP-6 bound to E- and L-sel with lower affinity ( Supplementary Fig. 19 ), consistent with reports of PSGL-1 binding to E- and L-sel at a K d of 2 to 5 μM (ref. 28 ). Sulfotyrosine exhibits poor stability under acid and near neutral conditions, thereby limiting its use in drug development. For example, rapid decomposition occurs at 37 °C on exposure to TFA and other scavengers used in peptide synthesis and the hydrolysis rate of sulfotyrosine increases with increasing temperature [42] , [43] . Consistent with these observations, the native N-terminal PSGL-1 sequence, GSP-6, rapidly degraded under low pH conditions (pH~5; T =37 °C). In contrast, the GS n P-6 mimic demonstrated superior stability when subjected to both low pH (pH~5; T =37 °C) and high temperature (pH7~7.5; T =60 °C), without observed degradation products as detected by RP-HPLC ( Fig. 2f ). Molecular dynamics simulations Computational simulations were used to predict key structural residues responsible for P-sel/GSnP-6 interactions. Molecular dynamics (MD) simulations were first validated by reproducing all structural attributes of the PSGL-1/P-sel interaction, as defined by crystallographic data and experimental investigations. The positions of the glycan and the peptide components of PSGL-1 were monitored over the course of simulating its interaction with P-sel ( Supplementary Fig. 20 ). Simulations confirmed that the ligand remained stable in the binding site, with the glycan displaying less positional variation than the peptide. In addition, all experimentally observed hydrogen bonds and salt bridges between the ligand and the protein were observed during the MD simulations. Of note, the dynamic motions of the system weakened some of these interactions relative to others ( Supplementary Table 2 ). In particular, while the hydrogen bonds associated with the glycan appeared markedly stable, the interactions between the tyrosine sulfate residues and the P-sel surface residues were relatively unstable and depended heavily on the protonation state of H114. This is consistent with a recent report by Cao et al. [45] , who demonstrated that the protonation state of H114 impacts the binding affinity of PSGL-1 to P-sel. As expected, full protonation of this histidine enhanced the stability of these interactions, particularly those associated with tyrosine sulfate (Y607) and H114. Similarly, the structure ( Fig. 3 ) and stability ( Supplementary Fig. 20 ) of GSnP-6 in the fully protonated H114 complex was comparable to that observed for the native PSGL-1 sequence, and retained all of the key non-covalent interactions ( Supplementary Table 1 ). In the case of neutral H114, the interactions between the tyrosine sulfonates and the protein were unstable, leading to orientation disruption of the peptide component in GSnP-6. The frequency of the rebinding interaction was too low to observe statistical convergence in the MD simulation ( Supplementary Fig. 20 ). Thus, only simulations with fully protonated H114 were employed in the subsequent analysis of interaction energies. 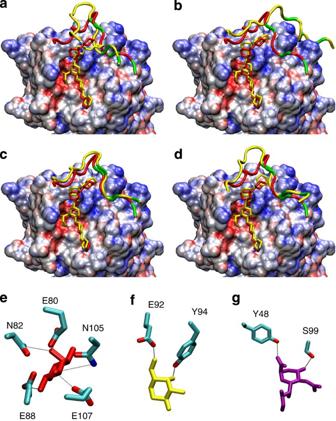Figure 3: Interactions of the N terminus of PSGL-1 and GSnP-6 bound to P-selectin, as a function of the protonation state of H114. Conformation of PSGL-1 (a) and GSnP-6 (b) ligands most similar to the average shape acquired from MD simulations performed with neutral H114. The crystal structure of the PSGL-1 ligand is shown in red with a splined representation of the peptide backbone, sulfated amino acid positions in green and a stick representation for monosaccharide rings. Assuming that H114 is fully protonated leads to optimal reproduction of the crystallographic data for PSGL-1 (c) and leads to similar binding for GSnP-6 (d). The solvent-accessible surface of P-selectin is coloured according to the electrostatic potential (acidic region: red; basic region: blue). (e–g) Hydrogen bonds between Fuc (red), Core-2Gal (yellow), and Neu5Ac (purple) and P-selectin residues. Figure 3: Interactions of the N terminus of PSGL-1 and GSnP-6 bound to P-selectin, as a function of the protonation state of H114. Conformation of PSGL-1 ( a ) and GSnP-6 ( b ) ligands most similar to the average shape acquired from MD simulations performed with neutral H114. The crystal structure of the PSGL-1 ligand is shown in red with a splined representation of the peptide backbone, sulfated amino acid positions in green and a stick representation for monosaccharide rings. Assuming that H114 is fully protonated leads to optimal reproduction of the crystallographic data for PSGL-1 ( c ) and leads to similar binding for GSnP-6 ( d ). The solvent-accessible surface of P-selectin is coloured according to the electrostatic potential (acidic region: red; basic region: blue). ( e – g ) Hydrogen bonds between Fuc (red), Core-2Gal (yellow), and Neu5Ac (purple) and P-selectin residues. Full size image Combinations of five GB parameterizations and protein dielectric constant values ( ε ) ranging from 1 to 5 were initially evaluated to determine which, if any, set of conditions reproduced the relative contributions of PSGL-1 constituent features to P-sel-binding affinity. Optimal conditions were then employed to assess the interaction energies of GSnP-6 with P-sel, as well as the contributions of distinct structural features of the analogue. The molecular mechanics-generalized born solvent-accessible surface area (MM/GBSA) calculations using either the GB 2 OBC or GB 1 OBC model produced comparable results with ε =4.0, in agreement with relative experimental values ( Supplementary Table 2 ). Since the GB 1 OBC parameterization has been successfully employed to compute interaction energies in other carbohydrate–protein systems involving charged moieties, it was selected over the GB 2 OBC parameterization ( Supplementary Fig. 21 ) [46] . This combination was able to correctly rank the relative contributions to binding, with Fuc≈total sulfate>Neu5Ac, and identified that the second sulfate made a larger contribution (by −1.3 to −1.6 kcal mol −1 ) than the other two. The experimental interaction energies of P-sel with PSGL-1 ligand and the analogue GSnP-6 were similar at −9.8 kcal mol −1 ( K d =73 nM) and −10.5 kcal mol −1 (22 nM), respectively. Using the combination of GB 1 OBC with ε =4.0, the absolute interaction energies of P-sel with PSGL-1 and GSnP-6 were predicted to be −45.1±3.4 kcal mol −1 and −44.6±3.1 kcal mol −1 , respectively ( Table 1 ). As anticipated, due to the omission of entropic penalties, predicted interaction energies were almost fourfold larger than experimental values [47] , [48] , [49] . Nonetheless, interaction energies were statistically equivalent, which is in agreement with experimental data. To facilitate detection on binding microarrays, GSnP-6 was chemically derivatized with a 7-amino-4-methylcoumarin (MCA) tag, which alters net charge, as well as local properties of the terminal lysine. The MCA tag was not included in the modelling, which employed only a lysine residue. The remaining residues in the peptide sequence of PSGL-1 and GSnP-6 render essentially identical contributions to the interaction energies. Due to the similarities of the two ligands, the relative contributions of the glycans to binding affinity were also indistinguishable within standard deviations. Likewise, the individual contributions from each sulfate group were comparable for each ligand, despite chemical differences ( Table 1 ). An unexpected and potentially significant observation concerns the second tyrosine sulfate residue (607), whose strong affinity (−8.4 to −9.5 kcal mol −1 ) appears to arise predominantly from van der Waals interactions (−6.6 to −7.0 kcal mol −1 ). In summary, computational analysis reproduced salient structural and energetic features of PSGL-1/P-sel interactions and predicted that GSnP-6 would behave comparably, consistent with observed affinity data ( Fig. 3 ). Table 1 Per-residue MM/GBSA interaction energies* for interactions of P-selectin with residues in PSGL-1 and GSnP-6. Full size table GSnP-6 inhibits P- and L-sel binding to PSGL-1 Flow cytometry was initially used to characterize the ability of GSnP-6 to block binding of sel Fc chimeras to murine and human leukocytes. Recombinant mouse P-, L- or E-sel-Fc chimera (2 μg ml −1 ) were incubated with murine leukocytes and GSnP-6 (0–30 μM). Likewise, recombinant human P-, L- or E-sel-Fc chimera (2 μg ml −1 ) were incubated with human peripheral blood leukocytes, as well as the human U937 cell line in the presence of GSnP-6 (0–30 μM). Binding of selectin chimeras was detected with phycoerythrin (PE)-conjugated anti-Fc antibody, quantified as mean fluorescent intensity and plotted as per cent inhibition. Specificity was confirmed with PSGL-1 blocking antibodies. GSnP-6 inhibited P-sel-dependent interactions in a dose-dependent manner in both human and mouse leukocytes, including human neutrophils (IC 50 ~14 μM), human monocytes (IC 50 ~20 μM), mouse neutrophils (IC 50 ~19 μM) and mouse monocytes (IC 50 ~28 μM) ( Fig. 4a,b ). GSnP-6 also inhibited PSGL-1/L-sel interactions at a somewhat lower potency (IC 50 ~30 μM) for human and mouse leukocytes ( Fig. 4c ). Inhibition of E-sel interactions was not observed over this concentration range ( Supplementary Fig. 22 ), which is consistent with the lower binding affinity of PSGL-1 for E-sel and the notion that leukocytes interact with E-sel through alternate ligands including CD44 and ESL-1 on mouse, and L-sel on human leukocytes [50] , [51] . 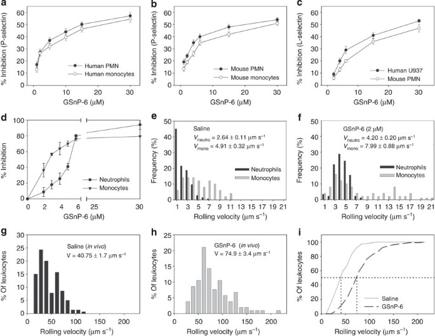Figure 4: GSnP-6 inhibits selectin adhesive interactionsin vitroandin vivo. (a,b) GSnP-6 (0–30 μM) was incubated with (a) human circulating PMN and monocytes or (b) mouse circulating PMN and monocytes and species appropriate P-selectin chimera, analyzed by flow cytometry and plotted as per cent inhibition versus PBS control. GSnP-6 inhibited P-selectin-dependent interactions in a dose-dependent manner in human and mouse leukocytes, including human neutrophils (IC50~14 μM), human monocytes (IC50~20 μM), mouse neutrophils (IC50~19 μM) and mouse monocytes (IC50~28 μM). (c) GSnP-6 inhibited PSGL-1/L-selectin interactions to human U937 and mouse neutrophils with a lower potency (IC50~30 μM). Data are represented as mean±s.e.m.,n=3. (d–f) GSnP-6 inhibits P-selectin/PSGL-1 adhesion under shearin vitro. (d) GSnP-6 (0–6 μM) exhibits dose-dependent inhibition of human neutrophil and human monocyte rolling and arrest on a recombinant ICAM-1/P-selectin substrate in the presence of shear;n=3 PBS,n=3 per GSnP-6 dose, velocities (μm s−1) of 120 cells per condition were measured, data are plotted as mean±s.e.m. (e,f) GSnP-6 increases rolling velocity of neutrophils and monocytes, cumulative frequency histograms are shown for PBS vehicle control (e) and 2 μM GSnP-6 (f);Vneutrophil: saline versus GSnP-6,P<0.0001 (Student’st-test);Vmonocyte: saline versus GSnP-6,P<0.0001 (Student’st-test). (g–i) GSnP-6 (4 μmol kg−1,n=4 mice, 5 leukocytes per vessel analyzed in 28 vessels) or saline control (n=3 mice, 5 leukocytes per vessel analyzed in 21 vessels) were delivered i.v. and leukocyte rolling velocity was recorded 15–25 min post surgical stimulation of the mouse cremaster to characterize P-selectin-dependent responsesin vivo;Vmean: saline versus GSnP-6,P<0.01 (Student’st-test). (i) Cumulative frequency histogram of leukocyte rolling velocities, median values indicated by vertical lines (median velocity saline=35.5 μm s−1, median velocity GSnP-6=64.0 μm s−1). Figure 4: GSnP-6 inhibits selectin adhesive interactions in vitro and in vivo . ( a , b ) GSnP-6 (0–30 μM) was incubated with ( a ) human circulating PMN and monocytes or ( b ) mouse circulating PMN and monocytes and species appropriate P-selectin chimera, analyzed by flow cytometry and plotted as per cent inhibition versus PBS control. GSnP-6 inhibited P-selectin-dependent interactions in a dose-dependent manner in human and mouse leukocytes, including human neutrophils (IC 50 ~14 μM), human monocytes (IC 50 ~20 μM), mouse neutrophils (IC 50 ~19 μM) and mouse monocytes (IC 50 ~28 μM). ( c ) GSnP-6 inhibited PSGL-1/L-selectin interactions to human U937 and mouse neutrophils with a lower potency (IC 50 ~30 μM). Data are represented as mean±s.e.m., n =3. ( d – f ) GSnP-6 inhibits P-selectin/PSGL-1 adhesion under shear in vitro . ( d ) GSnP-6 (0–6 μM) exhibits dose-dependent inhibition of human neutrophil and human monocyte rolling and arrest on a recombinant ICAM-1/P-selectin substrate in the presence of shear; n =3 PBS, n =3 per GSnP-6 dose, velocities (μm s −1 ) of 120 cells per condition were measured, data are plotted as mean±s.e.m. ( e , f ) GSnP-6 increases rolling velocity of neutrophils and monocytes, cumulative frequency histograms are shown for PBS vehicle control ( e ) and 2 μM GSnP-6 ( f ); V neutrophil: saline versus GSnP-6, P <0.0001 (Student’s t -test); V monocyte: saline versus GSnP-6, P <0.0001 (Student’s t -test). ( g – i ) GSnP-6 (4 μmol kg −1 , n =4 mice, 5 leukocytes per vessel analyzed in 28 vessels) or saline control ( n =3 mice, 5 leukocytes per vessel analyzed in 21 vessels) were delivered i.v. and leukocyte rolling velocity was recorded 15–25 min post surgical stimulation of the mouse cremaster to characterize P-selectin-dependent responses in vivo ; V mean: saline versus GSnP-6, P <0.01 (Student’s t -test). ( i ) Cumulative frequency histogram of leukocyte rolling velocities, median values indicated by vertical lines (median velocity saline=35.5 μm s −1 , median velocity GSnP-6=64.0 μm s −1 ). Full size image GSnP-6 inhibits leukocyte rolling and arrest PSGL-1 interactions with P-sel have been shown to signal activation of CD18 (β2-integrin) to adopt a high affinity extended conformation resulting in integrin-dependent deceleration and cell arrest. Inhibition of this interaction leads to an increase in rolling velocity and a reduction in cell arrest [51] . Human neutrophils and monocytes were incubated with GSnP-6 (0–30 μM) or PBS vehicle for 10 min and perfused through a microfluidic flow chamber at 2 dyn cm −2 over glass substrates coated with ICAM-1 and P-sel-Fc chimeras [52] . Total cell capture, defined as the number of cells that rolled or arrested (velocity ≤1 μm s −1 ), was determined, along with leukocyte rolling velocity. Videomicroscopic analysis demonstrated that GSnP-6 lead to a dose-dependent inhibition of monocyte and neutrophil capture in shear flow, with an IC50 of 3 μM and 5 μM, respectively ( Fig. 4d ). At a concentration as low as 2 μM, GSnP-6 increased the rolling velocity of human neutrophils and monocytes and resulted in 80% inhibition at 6 μM, a dose that abrogated the fraction achieving arrest ( Fig. 4d–f ). In contrast, incubation with the sulfated polysaccharide, fucoidan, at a concentration of up to 50 μg ml −1 (~50 μM) did not affect the efficiency of capture, rolling or arrest when compared with PBS control (data not shown). GSnP-6 at concentrations as high as 30 μM did not perturb leukocyte rolling and arrest on substrates coated with ICAM-1 and E-sel ( Supplementary Fig. 23 ). This implies that GSnP-6 specifically inhibits the interaction between PSGL-1 and P-sel in neutrophils and monocytes over this concentration range. Intravital microscopy was performed within 30 min of surgical stimulation of the murine cremaster muscle to determine the ability of GsnP-6 to inhibit leukocyte binding to microvascular endothelium in vivo [53] . Seven venules per mouse ( n =4, saline control; n =3, GSnP-6, 4 μmol kg −1 i.v.) with a diameter of 30–40 μm were analyzed and the velocities of 5–10 rolling leukocytes were determined in each venule by individually tracking leukocyte distance/time (μm s −1 ). A significant increase in mean rolling velocity was observed after intravenous administration of GSnP-6 when compared with saline vehicle control ( Fig. 4g,h , saline: 40.8±1.7 μm s −1 versus GSnP-6: 74.9±3.4 μm s −1 ; P ≤0.01; Student’s t -test). Cumulative frequency histogram analysis demonstrated a twofold increase in median rolling velocities ( Fig. 4i , saline: 35.5 μm s −1 versus GSnP-6: 64.0 μm s −1 ; Supplementary Fig. 24 ). GSnP-6 inhibits thromboinflammatory events in vivo PSGL-1/P-sel interactions are responsible for the formation of leukocyte–platelet aggregates, which promotes the infiltration of leukocytes, as well as the release of neutrophil extracellular traps and other procoagulant factors [54] . Human and murine platelet–leukocyte aggregates were quantified in whole blood using dual-label flow cytometry [55] . Human or mouse blood was stimulated with a thrombin receptor-activating peptide to induce platelet P-sel expression and dosed with 40 μM GSnP-6. GSnP-6 inhibited 65% of platelet–neutrophil and 72% of platelet–monocyte aggregate formation in human blood ( Fig. 5a,b ; P <0.05; Student’s t -test) and 42% of platelet–neutrophil and 47% of platelet–monocyte aggregate formation in murine blood ( Fig. 5c,d ; P <0.05; Student’s t -test). 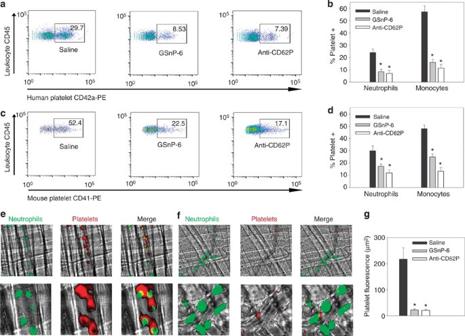Figure 5: GSnP-6 limits platelet–leukocyte aggregationin vitroandin vivo. (a–d) Anti-coagulated human or mouse blood was dosed with 40 μM GSnP-6 at room temperature and stimulated for platelet P-selectin expression with thrombin receptor-activating peptide (40 μM human PAR1-activating peptide, 200 μM mouse PAR4-activating peptide). Platelet–leukocyte aggregates were quantified by two-colour flow cytometry; CD45+monocyte and neutrophil populations were discerned through characteristic side scatter and quantified as % Platelet positive in saline control, 40 μM GSnP-6, and anti-CD62P (5 μg ml−1human KPL-1, 5 μg ml−1mouse RB40.34) treated samples. (a) Representative scatter plot of human samples incubated with anti-CD42a-PE and anti-CD45-APC, (b) % Platelet-positive neutrophils and monocytes in human samples, GSnP-6 inhibited 65% of platelet–neutrophil and 72% of platelet–monocyte aggregate formation in human blood. (c) Representative scatter plot of mouse samples incubated with anti-CD41-PE and anti-CD45-APC, (d) % Platelet-positive neutrophils and monocytes in mouse samples, GSnP-6 inhibited 42% of platelet–neutrophil and 47% of platelet–monocyte aggregate formation in mouse blood. Data representative of triplicate sample mean±s.e.m., *P<0.05 versus saline control (Student’st-test). (e–g)In vivoplatelet–leukocyte aggregation in a TNF-α model of venular inflammation. (e) Intravital microscopy of venular inflammation 3 h after administration of TNF-α demonstrates platelet aggregation and platelet–PMN binding after administration of saline control (PMN green; platelet red). (f) Platelet aggregation and platelet–PMN binding are not observed after administration of GSnP-6 (4 μmol kg−1iv). (g) The platelet inhibitory effect of GSnP-6 was equivalent to that observed for anti-CD62P, a P-selectin blocking antibody (75 μg per mouse i.v.) and was significantly less than saline control (*P<0.05 versus saline (Student’st-test),n=5 mice per treatment, 8–10 venules per mouse analyzed; error bars are represented as s.e.m.). Figure 5: GSnP-6 limits platelet–leukocyte aggregation in vitro and in vivo . ( a – d ) Anti-coagulated human or mouse blood was dosed with 40 μM GSnP-6 at room temperature and stimulated for platelet P-selectin expression with thrombin receptor-activating peptide (40 μM human PAR 1 -activating peptide, 200 μM mouse PAR 4 -activating peptide). Platelet–leukocyte aggregates were quantified by two-colour flow cytometry; CD45 + monocyte and neutrophil populations were discerned through characteristic side scatter and quantified as % Platelet positive in saline control, 40 μM GSnP-6, and anti-CD62P (5 μg ml −1 human KPL-1, 5 μg ml −1 mouse RB40.34) treated samples. ( a ) Representative scatter plot of human samples incubated with anti-CD42a-PE and anti-CD45-APC, ( b ) % Platelet-positive neutrophils and monocytes in human samples, GSnP-6 inhibited 65% of platelet–neutrophil and 72% of platelet–monocyte aggregate formation in human blood. ( c ) Representative scatter plot of mouse samples incubated with anti-CD41-PE and anti-CD45-APC, ( d ) % Platelet-positive neutrophils and monocytes in mouse samples, GSnP-6 inhibited 42% of platelet–neutrophil and 47% of platelet–monocyte aggregate formation in mouse blood. Data representative of triplicate sample mean±s.e.m., * P <0.05 versus saline control (Student’s t -test). ( e – g ) In vivo platelet–leukocyte aggregation in a TNF-α model of venular inflammation. ( e ) Intravital microscopy of venular inflammation 3 h after administration of TNF-α demonstrates platelet aggregation and platelet–PMN binding after administration of saline control (PMN green; platelet red). ( f ) Platelet aggregation and platelet–PMN binding are not observed after administration of GSnP-6 (4 μmol kg −1 iv). ( g ) The platelet inhibitory effect of GSnP-6 was equivalent to that observed for anti-CD62P, a P-selectin blocking antibody (75 μg per mouse i.v.) and was significantly less than saline control (* P <0.05 versus saline (Student’s t -test), n =5 mice per treatment, 8–10 venules per mouse analyzed; error bars are represented as s.e.m.). Full size image The capacity of GSnP-6 to inhibit early thromboinflammatory events in vivo was characterized by platelet adhesion to leukocytes and platelet aggregation in a cremaster model of tumour-necrosis factor-α (TNF-α)-induced venular inflammation [56] . TNF-α was administered intrascrotally (0.5 μg) to male mice (6–8 weeks old, C57BL/6) 3 h prior to imaging. P-sel blocking antibody (RB40.34), GSnP-6, or saline was subsequently administered at the time of imaging and platelet microaggregate formation and platelet–neutrophil binding was monitored in venules ( d 30–45 μm, 8–10 venules per mouse, n =5 mice per test group) over 2 min intervals through visualization of platelets and neutrophils labelled with Dylight 649-anti-CD42b and Alexa Fluor 488-anti-Gr-1 antibodies, respectively. Three hours after intrascrotal administration of TNF-α, venule endothelial cells display ~700 mm 2 adherent neutrophils and limited rolling flux (~1 white blood cells per min) ( Supplementary Fig. 25 ). Although administration of anti-CD62P or GSnP-6 at this stage would not be expected to alter established populations of adherent leukocytes, leukocyte–platelet interactions and platelet aggregate formation can be examined. Platelet accumulation was quantified by calculating median integrated fluorescence intensity, normalized to vessel surface area. GSnP-6 significantly reduced platelet–neutrophil interactions and platelet thrombi formation, similar to that observed after administration of a P-sel blocking antibody (* P <0.05, Student’s t -test; Fig. 5c ; Supplementary Fig. 25 ). The PSGL-1/P-sel pathway plays a critical role in disorders of innate immunity [12] , [17] , [57] , [58] , thrombosis [19] , [59] and cancer [60] , [61] and, as a consequence, the pharmacological blockade of this pathway represents an important therapeutic target. While the PSGL-1 glycan is a critical component of a diverse set of cell–cell recognition processes, as a complex glycoconjugate its recognition occurs in the context of other aglycone components that support leukocyte recruitment under shear stress of blood flow. Specifically, PSGL-1 is representative of a novel class of GSP that includes GPIbα [62] and endoglycan [63] , among many other important biomacromolecules. Detailed structural and mechanistic studies of PSGL-1 have revealed that high affinity recognition requires stereospecific interactions with both clustered tyrosine sulfates and a C2 O -glycan that bears a sLe x -containing hexasaccharide epitope [26] , [27] , [28] . Thus, while first generation small molecule inhibitors of P-sel/PSGL-1 interactions designed to mimic the sLe x moiety have proven valuable in validating targets, they have yet to achieve clinical benefit, which is likely related to their low binding affinity to selectins. Despite the potential of sLe x -GSPs, such as PSGL-1, to serve as tools for biological studies and the promise of PSGL-1 glycopeptide mimetics as therapeutic agents, their utility has been limited by low yield and limited stability. For example, synthesis of the C2 O -glycan typically suffers from suboptimal regioselectivity and may involve a triflic azide-mediated diazotransfer step, which is potentially explosive; thus, prohibiting preparative scale synthesis (>50 g). Likewise, the desire to generate clustered tyrosine sulfates by direct incorporation of Fmoc-Tyr (O-SO3-) amino acids during peptide synthesis is extremely challenging, owing to its acid lability. Alternatively, the sulfation of tyrosine residues by enzymatic sulfation is hindered by the instability of tyrosine sulfotransferase >20 °C and chemical sulfation is limited by low specificity, incomplete reaction and low yield. This report highlights three important milestones that effectively circumvent these problems. First, we have developed an efficient stereoselective route that has lead to multi-gram scale synthesis of the C2 O -glycan. This scheme is the shortest and most convenient reported to date, which has facilitated the synthesis of a broad range of GSP mimics. Second, we have determined that the acid labile Tyr (O-SO3-) moiety can be readily replaced with bioisosteric, hydrolytically stable Phe (p-CH2SO3H) and Phe (p-SO3H), increasing overall yield from <0.5 to 24%. The significance of these new synthetic strategies was demonstrated by the identification and production of a PSGL-1 glycopeptide mimic, GSnP-6, from a GSP library, which is very stable and has the highest affinity ( K d 22 nM) to P-sel reported to date. Our studies have confirmed that GSnP-6 potently blocks in a dose-dependent manner, the adhesion of platelet and leukocyte subsets implicated in the pathogenesis of variety of diseases. Finally, we have used GSnP-6 to establish a MD model as an important tool for providing new structural insights for the design and evaluation of additional novel PSGL-1 glycomimetics. In conclusion, a combination of chemical and enzymatic synthesis provided a diverse array of glycopeptide mimetics of PSGL-1. In the process, GSnP-6 was identified as a chemically stable compound that potently inhibits P-sel/PSGL-1 interactions both in the microvasculature and in model systems that reveal its antagonist specificity in blocking platelet, monocyte and neutrophil thromboinflammatory adhesion. A key discovery was the incorporation of stable sulfonated isosters, which permits facile peptide synthesis and provides a greater therapeutic window than the parent physiological ligand with considerable potential for application in disease states characterized by both acute and chronic inflammation. General All reagents were purchased from commercial sources and used as received, unless otherwise indicated. All solvents were dried and distilled by standard protocols. All reactions were performed under an inert atmosphere of argon or nitrogen, unless otherwise indicated. For peptide synthesis, Fmoc-Leu Novasyn TGA resin (resin loading: 0.3 mmol g −1 ), DMF (Biotech grade) and piperidine were purchased from Novabiochem. Fmoc-Phe(CH 2 SO 3 H)-OH and Fmoc-Phe(SO 3 H)-OH amino acids were purchased from RSP Amino Acids LLC. Coupling agents HBTU, HOBt and all other Fmoc-protected amino acids were purchased from EMD chemicals. Free reducing glycans, used as standards, were obtained from V-LABS Inc. (Covington, LA, USA). EZ-link NHS–biotin was purchased from Thermo Scientific (Rockford, IL, USA). Biotinylated lectins were from Vector Labs (Burlingame, CA, USA). Cyanine 5- and Alexa-488-labelled Streptavidin, Alexa488- and Alexa633-labelled secondary antibodies were purchased from Life Technologies (Woburn, MA, USA). Recombinant human ST3Gal IV and ST3Gal 1 were kind gifts from Dr Kelley Moremen at the University of Georgia. Studies with the anti-sulfotyrosine monoclonal antibody PSG2 were kindly performed with help from Dr Kevin Moore, Oklahoma Medical Research Foundation. Recombinant selectin Fc chimeras were purchased from R&D systems (Minneapolis, MN, USA). Protein A/G was purchased from Fischer Scientific (PI-21186). Fucoidan control was obtained from Sigma-Aldrich. The NHS-activated NEXTERION Slide H slides were purchased from Schott North America (Louisville, KY, USA). 1 H and 13 C were recorded with Inova 600 MHz spectrometer. High Resolution MALDI spectra were recorded by Harvard University Mass Spectrometry Center Waters Micro MX MALDI-TOF instrument. Optical rotation values were recorded using Perkin Elmer Polarimeter. All organic extracts were dried over sodium sulfate and concentrated under aspirator vacuum. All experimental protocols for compound synthesis, characterization data sets for all compounds, including NMR, HPLC and MALDI profiles, as well as details of computational and biological studies are provided in Supplementary Information . Microarray printing, binding assay and scanning For a multi-panel experiment on a single slide, the array layout was designed using Piezoarray software according to the dimension of a standard 14-chamber adaptor. The adaptor was applied on the slide to separate a single slide to 14 chambers sealed from each other during the experiment. All glycopeptides and control samples were printed on a NHS-activated glass slide in phosphate buffer (300 mM sodium phosphates, pH 8.5). The average spot volume was within 10% variation (intra-tip) of 0.33 nl. The average spot size was 100 μm. The following glycans were derivatized with 2-amino-N-(2-aminoethyl)-benzamide (AEAB) [64] : asialobiantennary N-glycan NA2 (Galβ1–4GlcNAcβ1–2Manα1–6(Galβ1–4GlcNAcβ1–2Manα1–3)Manβ1–4GlcNAcβ1–4GlcNAc), the 2,3-disiaylated biantennary N-glycan NA2,3 (Neu5Acα2–3Galβ1–4GlcNAcβ1–2Manα1–6(Neu5Acα2–3Galβ1–4GlcNAcβ1–2Manα1–3)Manβ1–4GlcNAcβ1–4GlcNAc), the 2,6-disialylated biantennary N-glycan NA2,6 (Neu5Acα2–6Galβ1–4GlcNAcβ1–2Manα1–6(Neu5Acα2–6Galβ1–4GlcNAcβ1–2Manα1–3)Manβ1–4GlcNAcβ1–4GlcNAc) and lacto-N-neo-tetraose (LNnT) (Galβ1–4GlcNAcβ1–3Galβ1–4Glc). These AEAB derivatives and biotin–NHNH 2 , all at 50 μM concentration were printed on the microarray as controls and reference standards. After printing, the slide was placed in a high moisture chamber at 50 °C and incubated for 1 h. The slide was subsequently washed and blocked with 50 mM ethanolamine in 0.1 M Tris buffer (pH 8.0) for 1 h, dried by centrifugation and stored desiccated at −20 °C prior to use. The binding assay was performed by incubating the slide with human or mouse P-, E- or L- selectin (5 μg ml −1 in calcium buffer (pH 8.0). Binding is Ca 2+ dependent and was quantitatively inhibited by addition of EDTA. Detection was accomplished using Alexa 488 goat anti-Human IgG (5 μg ml −1 ). The slide was subsequently washed (TSM Buffer, five times), centrifuged and analyzed with a Perkin Elmer ProScanArray microarray scanner equipped with four lasers covering an excitation range from 488 to 637 nm. The scanned images were analyzed using ScanArray Express software ( Supplementary Fig. 18 ). Biacore binding assay of PSGL-1 mimics Biotinylated GS (n) P-6 was first captured quantitatively on a streptavidin-coated sensor chip (GE Healthcare). Different amounts of P-, L- or E-sel-Ig were incubated in the wells (2.5–60 μg ml −1 ) and bound selectins were detected using fluorescently labelled anti-human IgG. PL1 and CHO131 (Santa Cruz, CA, USA) are mAbs that recognize the peptide sequence and C2 sLe x , respectively, which were used to confirm the immobilization step and to compare the relative amount of glycopeptides on the chip ( Supplementary Fig. 19 ). The bound mAbs and selectins were removed from the sensor chip by injecting 10 mM glycine-HCl, pH 2.0, and 50 mM EDTA, respectively, at 20 μl/min for 30 s. The kinetic parameters were obtained by plotting the curves using a 1:1 binding model provided by the Biacore evaluation software. At low GSnP-6 density (<5 response units (RU)), no plateau was observed even at highest concentrations of L- or E- Sel-Ig (60 μg ml −1 ). By contrast P-Sel (P-Sel-Ig), generated a saturated binding curve irrespective of the GsnP-6-coated densities used (<5–60 RU), indicating that affinity of P-Sel-Ig for GSnP-6 is less dependent on the density of the immobilized ligand. The comparison of GSnP’s densities (<5 RU versus 60 RU) indicate that binding of L- or E-Sel-Ig has ~25-fold lower affinity for the immobilized GSnP-6 than P-Sel-Ig. MD simulation studies Force field parameters for the oligosaccharide and SO 3 − moiety in the tyrosine sulfate (YS) and tyrosine sulfonate (YCS) residues were taken from the GLYCAM06 (version h) [65] parameter set, while those for the protein came from AMBER12 (ff99sb) [66] . Parameters for the linkage between the SO 3 − group and the amino acid side chains were approximated from existing terms in two parameter sets ( Supplementary Table 3 ). Ensemble-averaged partial atomic charges for the YS and YCS residues were developed according to the standard GLYCAM protocol [65] , from a collection of 300 snapshots extracted at 0.1-ns intervals from MD simulations (30 ns) performed in explicit solvent (TIP3P) for the zwitterionic forms of each amino acid. The initial coordinates for the charge calculations were based on the crystal structure of a monomer of the P-sel/PSGL-1 complex obtained from the Protein Data Bank (PDB entry code: 1G1S). The coordinates for the YCS residues were generated by replacing the phenolic oxygen atom in the YS residue with a methylene group. Molecular electrostatic potentials were computed at the HF/6–31G*//HF/6–31G* level with the Gaussian03 software package [67] , and restrained electrostatic potential charge fitting was performed using the RESP procedure with a restraint weight of 0.01. During charge fitting, the amino acid backbone charges were constrained to the standard values employed in ff99sb. The MD simulations were initiated with RESP charge sets computed for single conformations of each residue. The MD simulations were performed under nPT conditions (12 Å TIP3P water buffer in a cubic box, covalent bonds involving hydrogen atoms constrained using the SHAKE algorithm, a time step of 2 fs with heating from 5 to 300 K over a period of 50 ps controlled by the Berendsen thermostat). Prior to MD simulation, the systems were subjected to energy minimization under nVT conditions (500 steps steepest descent (sd), followed by 24,500 steps of conjugate-gradient minimization). Prior to simulation, water molecules and sodium ions in the crystal structure were removed, and the strontium ion substituted by magnesium, because parameters for strontium ion are not available in AMBER. Missing residue E604 was added to Y605 at the N terminus of the ligand using the LEaP module in AMBER12 with the backbone conformation copied from the E154-Y155 sequence. Sodium counter ions were added to each protein–glycopeptide complex to achieve neutrality using LEaP, prior to solvation with TIP3P water (8 Å buffer in an octahedral box). Energy minimization of the solvated complexes was performed in two steps under nVT conditions. Initially, the positions of water molecules and counter ions were minimized (500 steps sd followed by 24,500 steps conjugate gradient), during which all other solute atoms were restrained (100 kcal mol −1 Å 2 ). In the second step, all restraints were removed with the exception of those on the protein backbone, and the minimization cycle was repeated. Subsequently, heating to 300 K was performed over 50 ps (nVT) with a weak restraint (10 kcal mol −1 Å 2 ) on the backbone atoms of P-Selectin only. Systems were then equilibrated at 300 K for 0.5 ns (nPT ensemble, with the Berendsen thermostat) prior to production MD, under the same conditions (covalent bonds involving hydrogen atoms constrained using SHAKE, 2-fs time step). Production MD simulations were for 250 ns performed with the GPU implementation of PMEMD from AMBER12. In all MD simulations, a non-bonded cut-off of 8 Å was applied to van der Waals interactions, with long-range electrostatics treated with the particle mesh Ewald approximation, and mixed 1–4 non-bonded scale factors applied, as recommended for systems containing both carbohydrates and proteins (SCEE=SCNB=1.0 for the oligosaccharide and SCEE=1.2 and SCNB=2.0 for the protein) [65] . MM/GBSA calculations were carried out on 10,000 snapshots extracted evenly from the entire simulation trajectory using the single-trajectory method [68] with the MMPBSA.py.MPI module. The ability to correctly predict the relative per residue contributions to affinity is essential if the MM-GBSA calculations are to be employed in the rational design of inhibitors based on the PSGL-1 structure. There are several parameterizations of the GBSA model, none of which has been established as optimal for use in analyzing glycopeptide–protein binding. Further, estimating the affinity of PSGL-1/P-sel interactions faces the additional challenge of quantifying the potentially highly polarizing influence of multiple charge–charge interactions. In a non-polarizable classical force field, one approach for addressing this limitation is to employ an internal dielectric constant ( ε ) greater than unity in the MM-GBSA analysis. Again, as in the case of the GB approximation, no optimal value for ε has been reported for this type of interaction, although typical values <4.0 D. Last, entropic effects arising from changes in conformational flexibility may be estimated separately, but may require very long MD simulations to achieve convergence, and are frequently omitted when computing estimates of relative affinity [69] . Because of the novel nature of interactions involving YS and YCS, the suitability of five different GB implementations was examined, specifically: (1) the Hawkins, Cramer, Truhlar pairwise generalized Born model with parameters described by Tsui and Case (GB HCT model, igb=1); the modified GB model developed by Onufriev, Bashford and Case, with the following values for α , β and γ : GB 1 OBC ( α =0.8, β =0.0, γ =2.909125, igb=2) and GB 2 OBC ( α =1.0, β =0.8, γ =4.8, igb=5); the GB n models described by Mongan, Simmerling, McCammon, Case and Onufriev: GB n 1 , igb=7; GB n 2 , igb=8. In addition, six different internal dielectric ( ε ) values ( ε =1.0, 1.5, 2.0, 3.0, 4.0 and 5.0) were considered in the MM/GBSA calculations. Flow cytometry Flow cytometry was used to quantify binding inhibition of (P-, L-, E-) selectin chimeras to human and mouse leukocytes [58] . Heparinized whole mouse blood was collected via cardiac puncture under the approval of the Animal Care and Use Committee of Beth Israel Deaconess Medical Center (BIDMC). Normal human blood draws were collected in citrate under approval of the BIDMC Institutional Review Board. The human monocyte cell line U937 was obtained from ATCC and cultured according to supplied protocols. Cells were incubated with increasing concentrations of GSnP-6 (0–30 μM) and Fc chimeras of human or mouse P-, L-, and E-sel (R&D Systems, 2 μg ml −1 ) followed by PE-conjugated anti-Fc (1:100). The interaction of the selectins with mouse leukocytes, human leukocytes, or human U937 was analyzed by flow cytometry (BD LSR II) and quantified (FlowJo) as mean fluorescent intensity and plotted as per cent inhibition. PSGL-1 specificity was examined in the presence of blocking antibodies KPL-1 (anti-human PSGL-1) and 4RA10 (anti-mouse PSGL-1). Inhibition experiments were performed in triplicate. GSnP-6 inhibited binding of P- and L-sel-IgG chimeras in a dose-dependent manner. The P-sel inhibitor KF38789 was included as a reference compound. Inhibition of E-sel-IgG binding was not observed over the examined concentration range ( Supplementary Fig. 22 ). In vitro flow assay Recombinant human ICAM-1-Fc, P-sel-Fc, and E-sel-Fc were purchased from R&D Systems (Lot #: DLA0914011, FDA0913111, and BGU0413091 respectively). Neutrophils and monocytes were isolated from freshly collected human blood from healthy donors consented through an approved UC Davis institutional review board protocol. Whole blood was layered over neutrophil or mononuclear cell separation media, Polymophoprep, an Axis Shield formulation purchased from Cosmo Bio USA. After centrifugation myeloid cells were extracted and washed with 4-(2-hydroxyethyl)-1-piperazineethanesulfonic acid buffered salt solution. Coverslips were prepared as follows: 25 mm diameter, #1.5 glass coverslips were Piranha etched to remove organic molecules and to deposit hydroxyl group molecules on the surface. The etched coverslips were submerged in acetone with 1% 3-aminopropyltriethoxysilane (APTES) to add aminosilane groups. Recombinant human ICAM-1-Fc along with either P-sel-Fc or E-sel-Fc were absorbed at 5 μg ml −1 for 1 h prior to the experiment. Human neutrophils were suspended at a concentration of 10 6 cells per ml in 4-(2-hydroxyethyl)-1-piperazineethanesulfonic acid buffered salt solution and allowed to incubate for 10 min with PBS (vehicle control), 2, 3, 4, 5, 6 and 30 μM concentrations of GSnP-6. Treated cells were perfused through a microfluidic flow chamber at a calculated shear stress of 2 dyn cm −2 and cell motion recorded at three to five fields of view at 7.5 frames per s for 2 min along the centerline of the channel using a Matrox Meteor II and ImagePro Plus software to analyze cell kinetics. To further observe neutrophil behaviour, buffer was infused and images were collected at two additional locations along the channel. Rolling and arrested neutrophils were determined by tracking the cell centroid over 10 s increments utilizing MTrack2 software plugin for ImageJ. Neutrophils moving at a velocity of <1 μm s −1 were considered to be arrested. Intravital microscopy Surgical preparation of the mouse cremaster was performed as previously described. All experiments were performed in the BIDMC Center for Hemostasis and Thrombosis Research Core and were approved by the Animal Care and Use Committee of the BIDMC. Mice were anesthetized with an i.p. injection of ketamine HCl (125 mg kg −1 ), xylazine (12.5 mg kg −1 ) and atropine (0.25 mg ml −1 ), and placed on a 37 °C surgical blanket. The jugular vein was cannulated with PE 10 tubing to allow introduction of reagents, including GSnP-6 (4 μmol kg −1 in saline), saline vehicle control or 0.5 μm Dragon Green microspheres (Bangs Laboratories, Inc) for the measurement of centerline velocity. The trachea was intubated with PE90 to facilitate breathing. The cremaster muscle was exteriorized, pinned to the stage and superfused with thermocontrolled bicarbonate-buffered saline equilibrated with 5% CO 2 in N 2 . The surgical procedure was accomplished within 10 min. Microvessel data were obtained using an Olympus AX microscope with × 60 or × 40 water immersion objectives recorded with a Hamamatsu C9300-201/Gen III videoscope image intensifier interface. Coordinated image acquisition and offline data analyses were carried out using SlideBook software (Intelligent Imaging Innovations). At the termination of the experiment, blood was drawn via cardiac puncture and analyzed for complete blood count. Venules (30–40 μm in diameter) were observed 15 to 25 min after surgical stimulation of tissue to study P-sel-dependent rolling. Vessel diameter was measured using SlideBook ruler. Centerline blood flow velocity ( V cl ) was determined by measuring frame-to-frame displacement of single fluorescent microspheres in the centre of the vessel wall. Volumetric blood flow rate ( Q ) was calculated using the equation Q =( V cl × 0.625 × A cs ), where A cs is the cross-sectional area of the vessel ( πr 2 ) and 0.625 is an empirical correction factor. Wall shear rate ( γ w ) was calculated as γ w =2.12 × [(8 × 0.625 × V cl )/ D v )], where D v is the vessel diameter. Haemodynamic parameters are reported in Supplementary Table 4 . Recordings of each vessel were analyzed in brightfield for 30 to 60 s and leukocyte rolling flux was characterized as the number of leukocytes passing a plane perpendicular to the vessel axis ( Supplementary Fig. 24 ). Total leukocyte flux was determined as a product of systemic leukocyte concentration (cells per μl) and volumetric blood flow rate (μl s −1 ). Leukocyte rolling was characterized as the rolling flux fraction, which is the number of rolling leukocytes reported as a percentage of total leukocyte flux. Rolling velocity (μm s −1 ) was measured by tracking individual leukocyte translation over 2 s. Assessment of platelet–leukocyte aggregation in vitro Platelet–leukocyte aggregates were quantified in whole blood using dual-label flow cytometry [55] . Anti-coagulated human or mouse blood was incubated with 40 μM GSnP-6 at room temperature and stimulated with thrombin receptor-activating peptide (human PAR 1 -activating peptide 40 μM; mouse PAR 4 -activating peptide 200 μM) to induce platelet P-sel expression. Platelet–leukocyte aggregates were quantified by two-colour flow cytometry by incubating human samples with anti-CD42a-PE and anti-CD45-APC and mouse samples with anti-CD41-PE and anti-CD45-APC. CD45+ monocyte and neutrophil populations were discerned through characteristic side scatter and quantified as % Platelet positive in saline control, GSnP-6 (40 μM) or anti-CD62P (human KPL-1 (5 μg ml −1 ), mouse RB40.34 (5 μg ml −1 ) treated samples. Assessment of platelet–leukocyte interactions in vivo TNF-α was administered intrascrotally (0.5 μg) to male mice (6–8 weeks old, C57BL/6) 3 h prior to surgical preparation and imaging. Surgical preparation of the cremaster was performed, as described above. Agents were administered through the jugular cannula just prior to cremaster exposure and imaging, including saline vehicle control, GSnP-4 (4 μmol kg −1 ), anti-CD62P blocking antibody (clone RB40.34, 3 mg kg −1 ), anti-platelet Dylight 649-anti-CD42b (Emfret, 1 μl g −1 ) and Alexa Fluor 488 anti-Gr-1 (0.5 μg g −1 ). Microvessel data were obtained using an Olympus AX microscope with a × 60 water immersion objective recorded with a Hamamatsu C9300-201/Gen III videoscope image intensifier interface. Coordinated image acquisition and offline data analyses were carried out using SlideBook software. For each treatment condition, platelet accumulation was characterized as median integrated fluorescence plotted during a 2-min time interval from 5 mice (8–10 venules per mouse). The platelet signal was quantified as area under the curve for each individual capture, plotted against time and normalized to vessel surface area. Platelet aggregation and platelet–PMN binding is observed in saline control vessels while limited platelet signal is captured in GSnP-6- and anti-CD62P-treated animals ( Supplementary Fig. 25A–D ). Characterization of leukocyte–endothelial interactions at 3 h post-TNFα activation revealed minimal rolling flux and similar levels of adherent leukocytes between all groups ( Supplementary Fig. 25E,F ). How to cite this article: Krishnamurthy, V. R. et al. Glycopeptide analogues of PSGL-1 inhibit P-selectin in vitro and in vivo . Nat. Commun. 6:6387 doi: 10.1038/ncomms7387 (2015).